Directed evolution of prenylated FMN-dependent Fdc supports efficient in vivo isobutene production Isobutene is a high value gaseous alkene used as fuel additive and a chemical building block. As an alternative to fossil fuel derived isobutene, we here develop a modified mevalonate pathway for the production of isobutene from glucose in vivo. The final step in the pathway consists of the decarboxylation of 3-methylcrotonic acid, catalysed by an evolved ferulic acid decarboxylase (Fdc) enzyme. Fdc belongs to the prFMN-dependent UbiD enzyme family that catalyses reversible decarboxylation of (hetero)aromatic acids or acrylic acids with extended conjugation. Following a screen of an Fdc library for inherent 3-methylcrotonic acid decarboxylase activity, directed evolution yields variants with up to an 80-fold increase in activity. Crystal structures of the evolved variants reveal that changes in the substrate binding pocket are responsible for increased selectivity. Solution and computational studies suggest that isobutene cycloelimination is rate limiting and strictly dependent on presence of the 3-methyl group. The irrefutable harmful environmental effects and depleting reserves of fossil fuels have powered an extensive amount of research to seek sustainable alternatives for the production of petrochemicals, including the gaseous alkene isobutene [1] , [2] , [3] . Due to the favourable reactivity, isobutene is widely used as a building block for fuel additives, rubber, plastic and a broad range of fine chemicals. Over 10 million tons of isobutene are produced every year, primarily by steam cracking crude oil. Low levels of microbial production of isobutene were first detected in the 1980s [4] , [5] , [6] . More recently, isobutene production via a modified mevalonate (MVA) pathway using mevalonate diphosphate decarboxylase (MVD) to decarboxylate 3-hydroxyisovaleric acid was reported [7] and subsequently patented [8] (Fig. 1A ). Further studies highlighted a more efficient route using ﻿mevalonate-3-kinase (M3K, Picrophilus torridus ) that catalyses isobutene formation through an unstable phosphorylated intermediate [9] , [10] . The highest reported whole-cell isobutene production rate of 507 pmol min −1 g cells −1 was reached using E. coli engineered with M3K, however, this remains about 10 5 -fold lower than is economically viable [7] , [9] . The slow conversion could be surpassed by an alternative route, such as the more direct conversion of methylcrotonyl-CoA to isobutene through a combination of a thioesterase with a non-oxidative decarboxylase. The prenylated flavin (prFMN)-dependent ferulic acid decarboxylases (Fdc) catalyse reversible non-oxidative (de)carboxylation of a range of acrylic acids with extended conjugation [11] , [12] , [13] , [14] . Recently, a reversible 1,3-dipolar cycloaddition mechanism was conclusively shown to underpin catalysis in Aspergillus niger Fdc ( An Fdc) [11] , [15] , [16] , [17] . First, the cycloaddition of the substrate results in cycloadduct Int1 (Fig. 1B ). Decarboxylation occurs concomitantly with ring opening to form Int2 . Following the exchange of CO 2 with E282, protonation by E282 results in cycloadduct Int3 that releases the product through cycloelimination. Cycloadduct strain, mediated by a clash between the substrate R group and enzyme residues is key in ensuring reversible 1,3-dipolar cycloaddition [17] . Recent studies have shown rational engineering of An Fdc can expand substrate scope to include aromatic substrates such as naphthoic acid [18] . Crotonic acid was found to inhibit An Fdc by apparently irreversibly binding to the prFMN cofactor [17] . However, acrylic acid substrates lacking extended conjugation have rarely been reported in the wider UbiD enzyme family. Arguably, the natural UbiD substrate closest to 3-methylcrotonic acid is trans-anhydromevalonate 5-phosphate (tAHMP), which is decarboxylated by a  UbiD-decarboxylase from a ﻿hyperthermophilic archaeon Aeropyrum pernix in an alternative mevalonate pathway [19] . Both 3-methylcrotonic acid and tAHMP contain a secondary beta carbon and lack extended conjugation, however, the phosphate group in tAHMP may facilitate strain manipulation in cycloadduct intermediates. A recent communication describes a pathway for the production of butadiene in E. coli where the decarboxylation of cis,cis -muconic acid is catalysed by Fdc from Saccharomyces cerevisiae enhanced by rational design [20] . Fig. 1: Isobutene production via the modified mevalonate pathway utilizing Fdc for the last step. A Routes to isobutene via modified mevalonate pathways. Previously published mevalonate diphosphate decarboxylase (MVD) [7] and mevalonate-3-kinase (M3K) [9] produce isobutene via 3-hydroxyisovaleric acid. Fdc1, co-expressed with UbiX, catalyses the decarboxylation of 3-methylcrotonic acid to give isobutene. B Fdc decarboxylation reaction mechanism with 3-methylcrotonic acid in blue and common Fdc substrates with a conjugated R-group in red. First, the 1,3-dipolar cycloaddition of the substrate to prFMN iminium leads to the first pyrrolidine cycloadduct, Int1 . Decarboxylation and ring-opening forms the noncyclic alkene adduct Int2 . Protonation by a conserved glutamic acid residue yields the second pyrrolidine cycloadduct Int3 followed by cycloelimination to give the product. Full size image Herein, we report on discovery and optimization through directed evolution of Fdc decarboxylation activity with 3-methylcrotonic acid to produce isobutene. We seek to understand how a substrate lacking extended conjugation and bulk can be decarboxylated by Fdc, especially in view of the fact crotonic acid acts as an inhibitor of prFMN. We discuss the structural basis for an increase in activity and selectivity in Trichoderma atroviride Fdc ( Ta Fdc ) evolved by directed evolution. Surprisingly, the optimized variants remain unable to decarboxylate crotonic acid, suggesting that in the case of the substrate 3-methylcrotonic acid the single additional methyl group plays a key role in the cycloelimination process. Computational studies are used to rationalize the effect of the 3-methyl substitution on product formation. Initial screening of Fdc homologues Initial in vivo screening tested 15 UbiD homologues co-expressed with UbiX ( E. coli K-12) in E. coli for conversion of 3-methylcrotonic acid into isobutene as detected by gas chromatography. 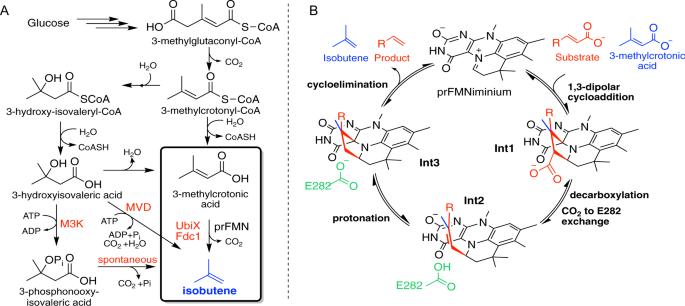Fig. 1: Isobutene production via the modified mevalonate pathway utilizing Fdc for the last step. ARoutes to isobutene via modified mevalonate pathways. Previously published mevalonate diphosphate decarboxylase (MVD)7and mevalonate-3-kinase (M3K)9produce isobutene via 3-hydroxyisovaleric acid. Fdc1, co-expressed with UbiX, catalyses the decarboxylation of 3-methylcrotonic acid to give isobutene.BFdc decarboxylation reaction mechanism with 3-methylcrotonic acid in blue and common Fdc substrates with a conjugated R-group in red. First, the 1,3-dipolar cycloaddition of the substrate to prFMNiminiumleads to the first pyrrolidine cycloadduct,Int1. Decarboxylation and ring-opening forms the noncyclic alkene adductInt2. Protonation by a conserved glutamic acid residue yields the second pyrrolidine cycloadductInt3followed by cycloelimination to give the product. Ta Fdc exhibited over twice the isobutene production compared to other homologues (Supplementary Table 1 ) and a directed evolution approach was taken to generate a variant of Ta Fdc with superior isobutene production activity and selectivity for 3-methylcrotonic acid over cinnamic acid (schematically presented in Supplementary Fig. 1 ). Ta FdcI, with a T405M mutation, was the first variant with a considerable increase in isobutene. Ta FdcV generated by 4 rounds of evolution has 11 mutations: E25N, N31G, G305A, D351R, K377H, P402V, F404Y, T405M, T429A, V445P and Q448W (Table 1 ). Characterization of Ta Fdc and Ta FdcV Ta Fdc wild-type and Ta FdcV with an N-terminal hexa-histidine tag were co-expressed with E. coli K-12 UbiX in E. coli and purified with Ni-NTA resin. UV–Vis spectra of both purified proteins exhibit a distinct peak at 380 nm, thought to correspond to the cofactor active form prFMN iminium (Supplementary Fig. 2A ) [16] . ESI-MS confirmed the presence of prFMN iminium in both enzyme variants (Supplementary Fig. 2B and C ). The shape of the 380 nm peak and cofactor content (assessed by the ratio of absorbances at 280 and 380 nm) varied from batch to batch. Ta Fdc showed decarboxylation activity with cinnamic and sorbic acid, with rates k obs = 7.2 ± 0.3 and 3.2 ± 0.3 s −1 , respectively (reported for a batch with a 380:280 nm ratio of 0.067). These values are comparable to those reported for An Fdc [11] , [16] . In contrast, the Ta FdcV variant showed compromised activity with sorbic acid ( k obs = 0.33 ± 0.03 s −1 ) and no activity was detected with cinnamic acid. When exposed to light, Ta Fdc sorbic acid decarboxylation activity steadily deteriorates with a half-life of 1 h compared to enzyme stored in dark (Supplementary Fig. 2H ). This is consistent with Fdc light-sensitivity as described previously [17] . Upon irradiation with a 405 nm LED lamp, the characteristic 380 nm peak in the UV–visible absorbance spectra of Ta Fdc and Ta FdcV irreversibly splits to peaks at 365 and 425 nm (Supplementary Fig. 2I and J ). Incubation of both Ta Fdc and Ta FdcV with 3-methylcrotonic acid triggered a change in the protein UV–Vis spectrum to reveal peaks at 340 and 425 nm, suggestive of a covalent substrate:prFMN adduct accumulating under turnover conditions. Following a desalting step, the spectrum returns to the as-isolated 380 nm single feature, confirming that a long-lived, inhibitory covalent complex with 3-methylcrotonic acid is not formed (Supplementary Fig. 2D and E ). Incubation of 80 μmol Ta FdcV with 10 mM 3-methylcrotonic acid led to a complete shift in the corresponding UV–Vis spectrum. In contrast, the wild-type Ta Fdc required prolonged incubation with 50 mM 3-methylcrotonic acid to achieve full spectral conversion, suggesting a substantially higher K D and/or adduct formation rate for the wild-type enzyme. An ESI-MS spectrum of the desalted sample showed peaks corresponding to both prFMN iminium and a putative Int3 prFMN cycloadduct with 3-methylcrotonic acid (Supplementary Fig. 3 ). This may be due to a small proportion of 3-methylcrotonic acid remains bound to prFMN as Int3 , suggesting Int3 elimination is the rate-limiting step, or that a proportion of the Int3 species has irreversibly isomerized to a more stable conformation. In order to assess the scope for activity with acrylic acids lacking extended conjugation, Ta Fdc and Ta FdcV were incubated with trans -2-pentenoic and trans -2-hexenoic acid, compounds that have previously been reported to undergo some An Fdc-mediated decarboxylation [11] . UV–Vis absorbance spectra indicated that Ta Fdc bound both acids (Supplementary Fig. 2F ), whereas the Ta FdcV variant preferred the smaller pentenoic acid and required higher concentrations to fully bind hexenoic acid (Supplementary Fig. 2G ). In contrast to samples incubated with 3-methylcrotonic acid, the UV–Vis spectra of samples incubated with pentenoic or hexenoic acid were unaffected by a desalting step, indicating that pentenoic and hexenoic acid irreversibly binds to Ta Fdc/ Ta FdcV. Quantitative GC assay indicates that pentene production from hexenoic acid by An Fdc is limited to a single turnover (Supplementary Fig. 4 ). Crystal structures of Ta Fdc and Ta FdcV reveal mutation impact on the substrate-binding pocket In order to understand how Ta FdcV mutations aid in isobutene production, crystal structures of Ta Fdc and Ta FdcV were solved at a resolution of 1.74 and 1.89 Å, respectively. An overlay of the wild-type and the variant crystal structures shows that the key residues F447, Q200 and the catalytic network of E287–R183–E292 are unaffected by the mutations (Fig. 2A ) [16] . The T405M mutation is located at the active site, extending towards the space above the prFMN uracil ring while the Q448W and F404Y mutations are situated in the second shell from the active site. The E292 residue side chain occupies ‘up’ and ‘down’ conformations, while weak electron density suggests a high degree of mobility for the L449 side chain. The mobile E292 and L449 gate access to the active site (Fig. 2B ) while the Q448W mutation in Ta FdcV narrows the binding pocket (Fig. 2C ). The T405M and Q448W mutations are likely to be responsible for the increased selectivity for 3-methylcrotonic acid in Ta FdcV by enhancing the substrate/active site shape complementarity, blocking access to larger substrates (Supplementary Fig. 5 ). While comparison of Ta Fdc and Ta FdcV crystal structures reveals the basis for increased selectivity in the evolved enzyme, it is not immediately clear why 3-methylcrotonic acid can yield isobutene from Int3 . Fig. 2: Comparison of Ta Fdc and Ta FdcV. A Two views of the overlay of Ta Fdc wild-type (green, 7NEY [10.2210/pdb7NEY/pdb]) and Ta FdcV (blue, 7NF0 [10.2210/pdb7NF0/pdb]) active sites. Comparison of Ta Fdc B and Ta FdcV C binding pockets. The mobile L449 and E292 gate the entrance to the active site and the Q448W mutation narrows the entrance to the active site. Full size image Formation of stable cycloadducts with inhibitors The effects of crotonic and 2-butynoic acid on Ta FdcV were studied to determine whether the mutations that increase in 3-methylcrotonic acid turnover also affected activity with related compounds. Incubation of Ta FdcV with 2-butynoic and crotonic acid led to the familiar split of the 380 nm prFMN peak in the UV–Vis spectrum (Fig. 3 A and D ), similar to 3-methylcrotonic acid. However, as previously observed with pentenoic and hexenoic acid, the spectrum did not recover the following desalting, suggesting that a covalent inhibitory adduct is formed. Similar trends were observed with Ta Fdc, however, incubation at higher inhibitor concentration was required to drive changes in the UV–Vis spectrum. Fig. 3: Cycloadduct formation in TaFdcV with inhibitors butynoic and crotonic acid. A UV–Vis spectra of Ta FdcV before and after incubating with 2-butynoic acid. B ESI–MS spectra of Ta FdcV incubated with 2-butynoic acid and desalted, showing the formation of prFMN-butynoic adduct [M + H] + = 607.18. C Crystal structure of Ta FdcV with prFMN-butynoic adduct (7NF1 [10.2210/pdb7NF1/pdb]). D UV–Vis spectra of Ta FdcV as is and incubated with crotonic acid E ESI–MS spectra of Ta FdcV incubated with crotonic acid (and desalted) showing the formation of decarboxylated prFMN-crotonic adduct [M–H] − = 565.21 and traces of prFMN-crotonic with the carboxylate group [M–H] − = 609.20. F Crystal structure of Ta FdcV prFMN-crotonic adduct (7NF2 [10.2210/pdb7NF2/pdb]). Full size image Upon addition of crotonic acid, a gradual shift in UV–Vis spectrum occurs over minutes, allowing estimation of adduct formation rate (Supplementary Fig. 6A ). The observed rate remains first order with respect to crotonic acid, with k obs = 0.34 ± 0.03 min −1 at the highest concentration tested (50 mM) (Supplementary Fig. 6B ). In contrast, a similar shift in UV–Vis spectrum upon addition of the substrate 3-methylcrotonic acid occurs rapidly within seconds, and at substantially lower 3-methylcrotonic acid concentrations. This suggests that crotonic acid adduct formation is hindered by a higher K D and/or slower rate of cycloaddition. ESI–MS and co-crystallization studies confirmed that the Ta FdcV 2-butynoic acid adduct stalls as Int1 , while the Ta FdcV crotonic acid adduct undergoes decarboxylation to stall at the Int3 species (Fig. 3 ). 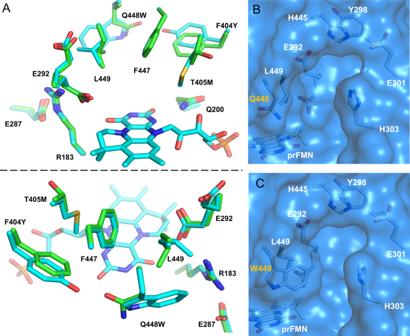Fig. 2: Comparison ofTaFdc andTaFdcV. ATwo views of the overlay ofTaFdc wild-type (green, 7NEY [10.2210/pdb7NEY/pdb]) andTaFdcV (blue, 7NF0 [10.2210/pdb7NF0/pdb]) active sites. Comparison ofTaFdcBandTaFdcVCbinding pockets. The mobile L449 and E292 gate the entrance to the active site and the Q448W mutation narrows the entrance to the active site. Similar behaviour has been reported for An Fdc [17] . No decarboxylation of the Int1 with 2-butynoic acid was detected, even in 1-month-old crystals. In contrast, although only Int3 was observed in co-crystals with crotonic acid, ESI-MS also showed a peak for the corresponding Int1 (Fig. 3E ). It is unclear whether Int1 can be detected in this case because decarboxylation of crotonic acid is slow, or because there is an equilibrium between Int1 and Int3 at ambient CO 2 levels. An FdcII with three point-mutations has an identical active site conformation to Ta FdcV To further understand how the architecture of the active site affects the decarboxylation of 3-methylcrotonic acid, corresponding key mutations from Ta FdcV were introduced in An Fdc. An Fdc has been established as a model system due to the fact that it readily yields atomic resolution crystal structures [11] , [16] , [17] , [18] . Two variants were studied: An Fdc T395M ( An FdcI) and the triple mutant An Fdc T395M R435P P438W ( An FdcII). Overlay of the An Fdc wild-type and Ta FdcV crystal structures reveals a downward shift of the Y404 residue in Ta FdcV in the secondary shell compared to the corresponding Y394 in An Fdc (Fig. 4A ). The Y394 residue is unaffected in the An FdcI variant compared to wild-type (Fig. 4B ). In contrast, the active site of the An FdcII variant matches that of Ta FdcV in the conformation of Y394 and M395 (Fig. 4C ). Fig. 4: Comparison of the TaFdcV and AnFdc wild-type and variant active sites. Overlay of Ta FdcV (green, 7NEY [10.2210/pdb7NEY/pdb]) with A An Fdc wild-type (blue, 4ZA4 [10.2210/pdb4ZA4/pdb]), B An FdcI (blue, 7NF3 [10.2210/pdb7NF3/pdb]) and C An FdcII (blue, 7NF4 [10.2210/pdb7NF4/pdb]) crystal structures ( An Fdc variant residue numbering according to An Fdc). Full size image As expected, neither An FdcI nor An FdcII were active with cinnamic acid, likely due to a clash between the substrate phenyl ring and M395. While binding of crotonic acid in An Fdc wild-type cannot be detected by the UV–Vis spectra over 2-h incubation, both mutants An FdcI and An FdcII readily bind the inhibitor, evident from UV–Vis spectra, demonstrating increased selectivity towards smaller substrates. Ta FdcII has comparable isobutene production activity to Ta FdcV Selected Ta Fdc variants (wild-type, Ta FdcI i.e. T405M, Ta FdcV, Ta FdcII, see Supplementary Fig. 1 ) and An Fdc variants (wild-type, An FdcI, An FdcII) were purified and assayed for isobutene production. Ta FdcII (F404Y, T405M, V445P, Q448W) was created by rational design based on the structural analysis of Ta Fdc wild-type, Ta FdcV and An FdcII. A comparison of the isobutene titre obtained following 2 and 4 h incubation revealed Ta FdcI and An FdcI produced 4–9 times the amount of isobutene compared to the wild-type enzymes. Additional mutations in An FdcII and Ta FdcII led to a substantial further increase of 18 and 81 fold, respectively, in isobutene production (Supplementary Fig. 7 ). Surprisingly, the in vitro titer obtained with Ta FdcII was slightly higher than the corresponding Ta FdcV levels obtained (Fig. 5 ). Thus, the 4 point mutations in Ta FdcII (F404Y, T405M, V445P, Q448W) and 3 point mutations in An FdcII (T395M, R435P, P438W), that create an active site architecture identical to Ta FdcV (Fig. 4 ), appear largely responsible for the increased isobutene activity compared to wild-type Ta Fdc and An Fdc. Fig. 5: Isobutene production by Ta Fdc and An Fdc variants. 3-methylcrotonate decarboxylation assay with purified enzyme comparing isobutene production as detected by GC by Ta Fdc and An Fdc variants (Table 1 ), both with N-terminal His-tags, over 2 and 4 h with 10 mM 3-methylcrotonate and 0.3 mg/mL enzyme. Fold increase comparison is shown in Supplementary Fig. 7 . Source data are provided as a Source Data file. Full size image While An Fdc wild-type was included in the initial UbiD screen, the An Fdc wild-type was 90 times lower in activity in vivo compared to Ta Fdc. Hence, An Fdc was not selected for further directed evolution, despite having comparable in vitro activity to Ta Fdc. The disparate and lower activity in vivo might be attributed to An Fdc-specific inhibition by metabolites such as phenylacetaldehyde [11] . An initial comparison of in vitro isobutene production levels using crude cell lysate from cells expressing Ta Fdc variants with those expressing MVD and/or M3K reveals a ~50-fold increase is observed for Ta FdcV compared to MVD/M3K levels (Supplementary Fig. 8 ). This demonstrates that the evolved Ta FdcV is vastly superior in catalysing the decarboxylative step compared to the previously described enzyme systems. Computational studies reveal a mechanistic basis for isobutene production It is curious that a single methyl group difference, as occurs between crotonic acid and 3-methylcrotonic acid, determines whether the compound is a substrate or inhibitor for the evolved Fdc variants. The marked influence of the additional methyl group on Int3 cycloelimination suggests this step may proceed via a cationic or radical beta carbon stabilized through additional hyperconjugation effects. A density functional theory (DFT) active site ‘cluster’ model (Supplementary Fig. 9 ) was used to investigate why 3-methylcrotonic acid is decarboxylated and eliminated by Ta FdcV in contrast to crotonic acid. The potential energy surface for the cycloelimination of Int3 to the non-covalent product complex was computed for both crotonic acid and 3-methylcrotonic acid by varying the C α –C 1’ and C β –C 4a bond lengths (Fig. 6 ). These suggest that 3-methylcrotonic acid undergoes a more asynchronous elimination, with the transition state C α –C 1’ and C β –C 4a bond lengths of 1.96 and 2.97 Å, respectively, compared to 1.95 and 2.77 Å for crotonic acid, respectively. This is linked to an increased charge separation occurring between the C β and prFMN for the 3-methylcrotonic acid compared to crotonic acid (Supplementary Tables 4 and 5 ), possibly affected by additional hyperconjugation in the case of 3-methylcrotonic acid. The release of propene from crotonic acid Int3 cycloadduct is more endothermic by ~8 kJ mol −1 and has a higher energy barrier by 19 kJ mol −1 compared to the release of isobutene from Int3 with 3-methylcrotonic acid. If the activation entropy is similar for the two reactions then the transition state energy difference translates to a ~2200 slower rate for the release of propene from Int3 at 293 K, explaining the lack of crotonic acid turnover under conditions tested. Fig. 6: DFT calculations applied to the active site of Ta Fdc with 3-methylcrotonic and crotonic acid. Contour map of the potential energy (kJ mol −1 ) landscape for 3-methylcrotonic acid ( A ) and crotonic acid ( B ) conversion to isobutene and propene, respectively, from Int3 by Ta FdcV, projected transition state is marked by X. C Zero-point energy corrected potential energy (kJ mol −1 , Supplementary Tables 2 and 3 ) scheme for 3-methylcrotonic (red) and crotonic acid (blue) with the Int3 set as 0 and the projected approximate transition state denoted with double daggers. D overlay of the DFT optimized transition states between Int3 and product for 3-methylcrotonic (pink, Cα–C 1’ and C β –C 4a bond lengths of 1.96 and 2.97 Å, respectively) and crotonic acid (blue, Cα–C 1’ and C β –C 4a bond lengths of 1.95 and 2.77 Å, respectively). Source data underlying A – C are provided as a Source Data file. Full size image The limit of prFMN-dependent (de)carboxylation by UbiD enzymes Directed evolution of Ta Fdc to Ta FdcV resulted in a marked increase in activity with 3-methylcrotonic acid. Surprisingly, the evolved mutant remained unable to convert crotonic acid to the corresponding propene. 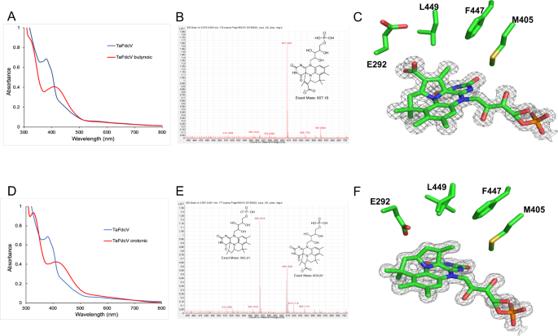Fig. 3: Cycloadduct formation in TaFdcV with inhibitors butynoic and crotonic acid. AUV–Vis spectra ofTaFdcV before and after incubating with 2-butynoic acid.BESI–MS spectra ofTaFdcV incubated with 2-butynoic acid and desalted, showing the formation of prFMN-butynoic adduct [M + H]+= 607.18.CCrystal structure ofTaFdcV with prFMN-butynoic adduct (7NF1 [10.2210/pdb7NF1/pdb]).DUV–Vis spectra ofTaFdcV as is and incubated with crotonic acidEESI–MS spectra ofTaFdcV incubated with crotonic acid (and desalted) showing the formation of decarboxylated prFMN-crotonic adduct [M–H]−= 565.21 and traces of prFMN-crotonic with the carboxylate group [M–H]−= 609.20.FCrystal structure ofTaFdcV prFMN-crotonic adduct (7NF2 [10.2210/pdb7NF2/pdb]). This contrasts with previous evolved studies aimed at expanding the An Fdc substrate repertoire to include (hetero)aromatic compounds [18] . In this case, the evolution of activity against heteroaromatic bicyclic compounds yielded a broad specificity variant able to convert even naphthoic acid. 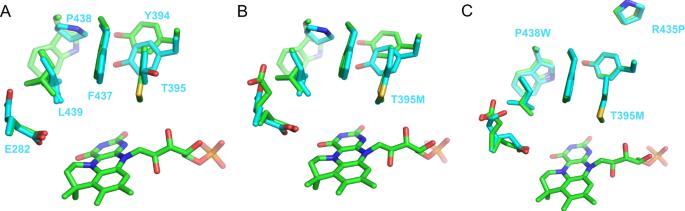Fig. 4: Comparison of the TaFdcV and AnFdc wild-type and variant active sites. Overlay ofTaFdcV (green, 7NEY [10.2210/pdb7NEY/pdb]) withAAnFdc wild-type (blue, 4ZA4 [10.2210/pdb4ZA4/pdb]),BAnFdcI (blue, 7NF3 [10.2210/pdb7NF3/pdb]) andCAnFdcII (blue, 7NF4 [10.2210/pdb7NF4/pdb]) crystal structures (AnFdc variant residue numbering according toAnFdc). It is thus possible that 3-methylcrotonic acid represents a limit for bona fide UbiD-substrates, indicating that prFMN-dependent catalysis requires more than an α , β -unsaturated acrylic acid (i.e. a secondary C β carbon) to yield reversible cycloelimination. Indeed, crotonic acid readily forms irreversible adducts with (evolved) Fdc that proceed to the last step prior to product formation. Detailed studies of the An Fdc mechanism revealed considerable enzyme-induced strain in substrate-cofactor adducts that avoid dead-end local energy minima during the covalent catalysis [17] . In the case of smaller substrates such as (3-methyl) crotonic acid, the scope for enzyme-induced strain as a tool to optimize the energy landscape is minimal. In this case, cycloelimination of isobutene appears feasible at ambient conditions whereas propene production is not. 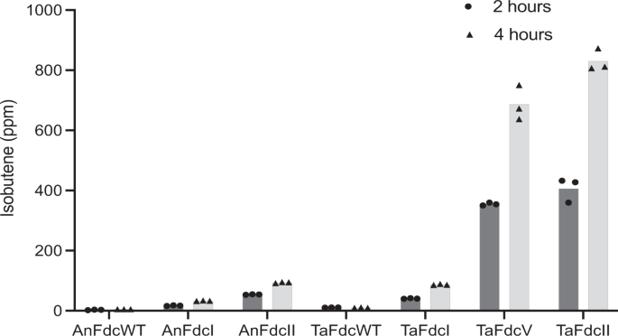Fig. 5: Isobutene production byTaFdc andAnFdc variants. 3-methylcrotonate decarboxylation assay with purified enzyme comparing isobutene production as detected by GC byTaFdc andAnFdc variants (Table1), both with N-terminal His-tags, over 2 and 4 h with 10 mM 3-methylcrotonate and 0.3 mg/mL enzyme. Fold increase comparison is shown in Supplementary Fig.7. Source data are provided as a Source Data file. Computational studies provide a rationale behind these observations, suggesting a ~2200 fold slower rate for the release of propene from Int3 . Thus, further optimization of isobutene production and future evolution of propene producing Fdc variants will need to focus on the energetics of the hydrocarbon elimination step. In vivo isobutene assay In vivo screenings were carried out on a 96-well plate (DW96, 2.2 mL wells, sealed with a foil sheet). Ta Fdc and other UbiD homologues were co-expressed with UbiX ( E. coli , K-12) in a petDuet vector (UbiD in MCS1 and UbiX in MCS2) in E. coli (BL21, DE3). Isobutene production from 0.4 mL reaction mix with 10 mM 3-methylcrotonic acid was detected from the headspace by gas chromatography. The GC method consisted of 100 µL of headspace with a split ratio of 10 injected to RTX-1 column (15 m, 0.32 mm internal diameter, 5 µm film thickness, from RESTEK 10178-111) using nitrogen as a carrier gas (1 mL/min flow rate). The oven temperature was held at 100 °C and the injector and detector were maintained at 250 °C. Isobutene was calibrated at 1000, 5000 and 10,000 ppm with standards from Messer. 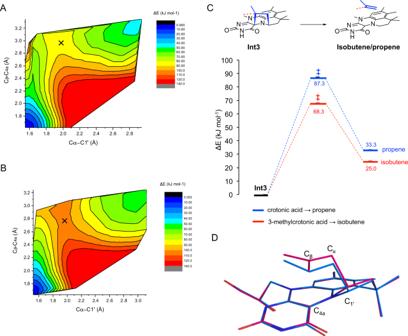Fig. 6: DFT calculations applied to the active site ofTaFdc with 3-methylcrotonic and crotonic acid. Contour map of the potential energy (kJ mol−1) landscape for 3-methylcrotonic acid (A) and crotonic acid (B) conversion to isobutene and propene, respectively, fromInt3byTaFdcV, projected transition state is marked by X.CZero-point energy corrected potential energy (kJ mol−1, Supplementary Tables2and3) scheme for 3-methylcrotonic (red) and crotonic acid (blue) with theInt3set as 0 and the projected approximate transition state denoted with double daggers.Doverlay of the DFT optimized transition states betweenInt3and product for 3-methylcrotonic (pink, Cα–C1’and Cβ–C4abond lengths of 1.96 and 2.97 Å, respectively) and crotonic acid (blue, Cα–C1’and Cβ–C4abond lengths of 1.95 and 2.77 Å, respectively). Source data underlyingA–Care provided as a Source Data file. Mutagenesis Point mutations ( Ta FdcI, Ta FdcII, An FdcI, An FdcII, Supplementary Table 6 ) were generated with a Q5 mutagenesis kit from New England Biolabs. Primers were designed with NEBaseChanger (New England Biolabs). The presence of the point mutation was confirmed by sequencing (Eurofins). Protein expression A pETDuet-1 vector containing genes for T. atroviride Fdc (with an N-terminal 6-histidine affinity tag) and UbiX ( E. coli , K-12) was transformed into BL21(DE3) competent cells following the manufacturer’s protocol (Novagen). A colony was inoculated into Lysogeny Broth (supplemented with 100 µg/mL ampicillin) and incubated by shaking overnight at 37 °C. 5 mL of LB culture was inoculated into 1 L of Terrific Broth (TB, Formedium), supplemented with 100 µg/mL ampicillin. The culture was incubated by shaking at 37 °C until the optical density of 0.6–0.8. The cells were induced with 0.4 mM isopropyl β- d -1-thiogalactopyranoside (IPTG) and supplemented with 0.5 mM MnCl 2 . The cultures were incubated by shaking at 18 °C for 24 h. The cells were harvested by centrifugation (10 min, 8939 × g ) and frozen. Protein purification Frozen cells were supplemented with EDTA-free protease inhibitor mixture (Roche Applied Science), lysozyme, DNAse, and RNAse (Sigma) and resuspended (50 mM HEPES, 300 mM KCl, pH 6.8). The cells were lysed by sonication on ice (Bandelin Sonoplus sonicator, TT13/F2 tip, 30% power with 20 s on/40 s off for 15 min) and centrifuged (1 h, 174,000–185,500 × g , Beckman Optima LE-80k ultracentrifuge, ﻿Ti50.2 rotor). The cell-free extract was loaded on Ni-NTA resin, washed with 4 column volumes of 40 mM imidazole buffer (40 mM imidazole, 50 mM HEPES, 300 mM KCl, pH 6.8) and eluted in 1 mL fractions with 250 mM imidazole buffer (250 mM imidazole, 50 mM HEPES, 300 mM KCl, pH 6.8). Fractions containing protein were combined and desalted into 25 mM HEPES, 150 mM KCl, pH 6.8. Exposure to light was minimized by covering with foil and using black Eppendorf tubes. Cycloadduct formation Ta FdcV (500 µL, 0.45 mM protein, 25 mM HEPES, 150 mM KCl, pH 6.8) was incubated with crotonic or 2-butynoic acid. The formation of the prFMN-crotonic acid cycloadduct was followed by UV–Vis spectroscopy and additional acid were added until full conversion (complete loss of the 380 nm peak). The protein was desalted to 25 mM HEPES, 150 mM KCl, pH 6.8 and plated for crystal trials. Crystallization and X-ray structure determination Crystallization was performed by sitting-drop vapour diffusion. Screening of 0.3 μL of 1 mg/mL Ta FdcV in 25 mM HEPES, 150 mM KCl, pH 6.8, and 0.3 μL of reservoir solution at 4 °C resulted in a number of hits in the BCS plate from molecular dimensions. Seed stocks were used to reproduce Ta Fdc wild-type crystals and co-crystals with 2-butynoic and crotonic acids in the BCS plate. Crystals were cryoprotected with PEG200 and flash-frozen in liquid nitrogen. An Fdc wild-type and variants were crystallized in 0.2 M potassium thiocyanate, Bis–Tris propane 6.5, 20% w/v PEG 3350 at 4 °C [16] . Diffraction data were collected at Diamond beamlines and processed using the CCP4 [21] suite version 7.1 (Supplementary Table 7 ). Phaser MR version 2.8.3 was used to perform molecular replacement using 4ZA4 [ https://doi.org/10.2210/pdb4ZA4/pdb ] as a model. Refinement was carried out with REFMAC5 [22] and manual rebuilding in COOT [23] version 0.9.5. Ligand definitions and coordinates were generated with AceDRG [24] . In vitro isobutene assay comparing Ta Fdc and An Fdc variants All variants were grown in BL21(DE3) cells with a pETDuet plasmid with the Fdc variant (N-terminal 6-His-tag) in the first multiple cloning site and UbiX (untagged, wild-type from E. coli K12) in second multiple cloning site. The cells were grown in a ZYM-5052 autoinducing medium (30 °C for 6 h, followed by 18 °C for 24 h). The Fdc variants were purified with Protino ® Ni-IDA column and stored at −80 °C (in 50 mM Tris–HCl pH 7.5, 1 mM MnCl 2 , 20 mM NaCl, 200 mM KCl, 10% glycerol). Decarboxylation of 3-methylcrotonate was set up in triplicates in 50 mM Tris–HCl pH 7.5, 1 mM MnCl 2 , 20 mM NaCl, 200 mM KCl with 10 mM 3-methylcrotonate and 0.3 mg/mL enzyme in DW384 plates (40 µL per well, sealed with foil sheet). Isobutene production was measured from headspace by gas chromatography after 2 and 4 h. In vitro isobutene assay comparing Ta Fdc, Sc MVD and Pt M3K An equal amount of E. coli cells containing either empty pETDuet (as control) or one of the following plasmids: pETDuet TaFdc_UbiX, pETDuet TaFdcV_UbiX, pETDuet PtM3K ( P. torridus mevalonate 3-kinase, Uniprot: Q6KZB1), pETDuet ScMVD ( S. cerevisiae MVD, Uniprot: P32377) or pETDuet PtM3K—ScMVD, were lysed in 50 mM Tris–HCl pH 7.5, 20 mM KCl, 2 mM MgCl 2 , 1 g/L lysozyme, 0.03 g/L DNAse for 1 h at 37 °C. A total of 150 μL of lysate was transferred to a 2 mL GC-vial and MgCl 2 (10 mM final concentration) was added. Substrates were added to 50 mM final concentration and 200 μL total volume, and consisted of either 3-hydroxyisovalerate/ATP, 3-phosphonooxy-isovalerate/ADP or 3-methylcrotonate. Following 4 h of incubation at either 37 or 50 °C, the reaction mixture was inactivated by incubation at 90 °C for 5 min. GC analysis of the gas phase was carried out as described above to determine isobutene levels produced. All reactions were carried out in duplicates. DFT calculations Ta FdcV active site cluster model with crotonic (365 atoms) and 3-methylcrotonic acid (368 atoms) was built based on the Ta FdcV crystal structure with crotonic acid bound as Int3 adduct (Supplementary Fig. 9 ) and modelled at the B3LYP/6–31 G( d , p ) level of theory with the D3 version of Grimme’s dispersion with Becke–Johnson damping and a generic polarizable continuum with ε = 5.7 using the polarizable continuum model [25] . C α –C 1’ and C β –C 4a bonds were both fixed for any single DFT optimization and substrate release was modelled using Gaussian 09 revision D.01. by lengthening one bond by 0.05 Å at a time, resulting in a 3D energy landscape consisting of ~900 DFT optimized models (for 3-methylcrotonic acid). Table 1 Summary table of An Fdc and Ta Fdc variants. Full size table Reporting summary Further information on research design is available in the Nature Research Reporting Summary linked to this article.